Clkpost-transcriptional control denoises circadian transcription both temporally and spatially The transcription factor CLOCK (CLK) is essential for the development and maintenance of circadian rhythms in Drosophila . However, little is known about how CLK levels are controlled. Here we show that Clk mRNA is strongly regulated post-transcriptionally through its 3′ UTR. Flies expressing Clk transgenes without normal 3′ UTR exhibit variable CLK-driven transcription and circadian behaviour as well as ectopic expression of CLK-target genes in the brain. In these flies, the number of the key circadian neurons differs stochastically between individuals and within the two hemispheres of the same brain. Moreover, flies carrying Clk transgenes with deletions in the binding sites for the miRNA bantam have stochastic number of pacemaker neurons, suggesting that this miRNA mediates the deterministic expression of CLK. Overall our results demonstrate a key role of Clk post-transcriptional control in stabilizing circadian transcription, which is essential for proper development and maintenance of circadian rhythms in Drosophila . Most organisms use circadian clocks to keep temporal order and anticipate daily environmental changes. Circadian clocks appear to function on a cell-autonomous basis and are generated by interconnected complex transcriptional and post-translational feedback loops [1] . In Drosophila , the master genes Clock ( Clk ) and cycle ( cyc ) activate the circadian system by promoting rhythmic transcription of a number of key genes [2] , [3] , [4] . Three of these target gene products, PERIOD (PER) [5] , TIMELESS (TIM) [6] and CLOCKWORK ORANGE (CWO) [7] , [8] , [9] , repress CLK-CYC-mediated transcription on a daily basis. CLK activates transcription only while associated with CYC. The latter is constitutively expressed, whereas CLK is present in limiting amounts [4] , [10] . The CLK-CYC heterodimer also activates the expression of VRILLE (VRI) and PAR-DOMAIN-PROTEIN 1 (PDP1), which have been postulated to be responsible for the oscillation of Clk mRNA [11] , [12] . Although the role of VRI in repressing Clk transcription is well established, recent reports suggest that PDP1 might not directly regulate Clk [13] . In addition to transcriptional control, post-transcriptional and post-translational regulations play also a central role in circadian timekeeping (for reviews see refs 14 , 15 , 16 ). Circadian clocks are widespread through the fly body [17] . However, a group of ∼ 150 neurons in the brain drives circadian rhythms in locomotor activity [18] . These neurons have been divided into several subgroups based on their anatomical location and expression of the core clock genes [19] , [20] . These groups are small and large ventral lateral (sLNvs and lLNvs), dorsal lateral (LNds), and dorsal (DN1s, DN2s and DN3s) neurons. The neuropeptide pigment dispersing factor (PDF), which is expressed exclusively in the LNvs, is essential for normal circadian patterns of activity in light and dark and for persistent circadian rhythms in constant darkness (DD) [18] . Despite the central role of Clk in the circadian system, it is still not well understood how CLK levels and activity are controlled. The current model states that most (if not all) of this control is through post-translational regulation such as phosphorylation, ubiquitination and other types of modifications [21] , [22] , [23] , [24] , [25] . Indeed, although Clk mRNA levels display strong transcriptional oscillations [11] , [12] , CLK protein levels are nearly constant though the day [26] . Moreover, expression of CLK under the tim or per promoter in ClkARK fly strains (in which transcription has the opposite daily phase relative to that under control of the Clk promoter [21] ) does not disrupt circadian behaviour, indicating that flies can adapt or compensate for high levels of CLK [21] . As these experiments were performed in a wild-type background, whether constant or shifted Clk transcription alone can drive circadian behavioural rhythms was not determined. In addition, it is well established that the levels or activity of CLK markedly alter the circadian period and amplitude [27] , [28] , [29] . Moreover, uncontrolled expression of CLK leads to death. For example, expression of CLK using the circadian driver tim -gal4 leads to embryonic lethality [30] , and induction of CLK-driven transcription using the CLKGR system results in adult death (Ron Weiss, personal communication). Some of the toxic effects of CLK overexpression are likely due to a central role of Clk in cell determination. Indeed, CLK expression in non-circadian cells is enough to generate ectopic circadian clocks in the fly brain [30] . In addition, CLK-driven transcription may have a role in the development of the circadian system, as Clk and cyc fly mutants display abnormalities in the morphology of circadian neurons [29] , [31] . These data demonstrate that post-translational control alone may not be enough to buffer big changes in CLK levels. Indeed, post-transcriptional regulation might also be important, as we demonstrated in the past that Clk is strongly regulated by miRNAs [32] . In brief, Clk is strongly bound to AGO1 and the miRNA bantam can regulate Clk levels in Drosophila S2 cells [32] . Moreover, we showed that the putative bantam binding sites on Clk 3′ UTR are essential for normal circadian rhythms [32] . However, how this regulation influences CLK levels and activity in time and space is still unknown. Circadian clocks are extraordinarily robust systems; they are able to keep time accurately without any timing cues. This robustness is likely the result of multiple layers of regulation that assure accurate timekeeping by buffering stochastic changes of clock-relevant activities. For example, it has been proposed that the main function of the redundancy and interlocked transcriptional feedback loops of the circadian system is to provide robustness to circadian transcription [33] , [34] , [35] , [36] . These layers of regulation extend even beyond the single-cell level. Circadian neurons in the brain are organized in a network that synchronizes and likely amplifies the individual neuronal oscillators thereby contributing to a coherent and robust behavioural output [2] , [37] , [38] , [39] . Circadian clocks must also control or buffer transcriptional noise and its consequences, especially for genes that are expressed at limiting levels (that is, Clk ), as it is well known that transcriptional noise is inversely correlated with transcriptional rate [40] . Here we demonstrate that the Clk 3′ UTR sets a threshold for meaningful circadian gene expression. Flies in which Clk is expressed without post-transcriptional control ( ClkSV40 flies) have ectopic circadian cells in the brain. Surprisingly the levels of CLK per cell are normal in these flies, indicating that Clk post-transcriptional regulation does not control the overall CLK levels. Interestingly, ClkSV40 flies have aberrant circadian transcription and behaviour, as well as widespread expression of CLK-target gene products in the brain. These behavioural deficits are accompanied by the vary stochastic development of pdf ->expressing LNvs cells that vary in number between individuals and even between the two lobes of the same brain. Similarly, flies carrying Clk transgenes with deletions in the binding sites for the miRNA bantam display stochastic number of pacemaker neurons, strongly suggesting that this miRNA is the key factor mediating the deterministic expression of CLK. We backed up this role for post-transcriptional control by a mathematical model that predicts the central role of Clk mRNA turnover in minimizing noise of the circadian feedback loops. All together, our results demonstrate that post-transcriptional control of a master transcriptional regulator is an efficient way of assuring deterministic transcriptional responses. Clk mRNA is under strong post-transcriptional control We recently showed that Clk mRNA levels are regulated by microRNAs (miRNAs) [32] . To address the importance of Clk post-transcriptional regulation, we compared Clk mRNA levels with those of other circadian mRNAs using previously published microarray and RNA-seq data from fly heads and brains [7] , [41] , [42] . In these data sets Clk mRNA levels were the lowest of the core circadian components ( Fig. 1a , Supplementary Fig. 1a,b ). 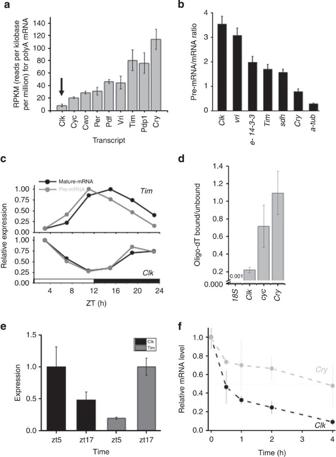Figure 1:Clkis under strong post-transcriptional regulation (a) Comparison of clock transcript levels. RNA-seq data41were used to compare expression levels of core circadian components in fly heads; an average of six timepoints±s.e. in LD conditions (ZT 2, 6, 10, 14, 18, 22) were analysed. (b) The levels of pre-mRNA and mRNA of core clock components were measured by real-time PCR (RT-PCR) from a mixture of six circadian time points and scaled using an equimolar mixture of the PCR products to obtain absolute measurements between the different mRNAs or pre-mRNAs in each sample (mean±s.e.; three biological replicas). As the values in each sample (pre-mRNA and mRNA) are normalized, the pre-mRNA/mRNA ratio is relative, not absolute (see methods for details). (c) RT-PCR measurements of transcriptional (grey) and steady state (black) levels ofClkandtim. Transcriptional/pre mRNA transcripts were detected using primers for intronic sequences of the genes, whereas steady-state/mature mRNAs were detected using primers flanking two exons. Expression was normalized to RP49 and rpS18. Representative experiment of three repeats is shown. (d) RT-PCR results presenting the ratio of mRNA bound to oligo-dT beads versus unbound mRNA. Data pooled from a mixture of six time points (mean±s.e.; three biological replicates). (e) ADrosophilafly wing system was developed to monitor circadian gene mRNA expression levels (normalized to RP49 at ZT5, 17).Clkandtimlevels cycle with the expected phase. The measurements were performed in triplicates for each time point using the Canton-S strain. (f) RT-PCR mRNA half-life measurements forClkandcrymRNAs from fly wings treated with actinomycin D in five different time points (0–4 h after actinomycin D exposure, 12 h light/12 h dark conditions,mean±s.e.; three biological replicates). See alsoSupplementary Fig. 1. Figure 1: Clk is under strong post-transcriptional regulation ( a ) Comparison of clock transcript levels. RNA-seq data [41] were used to compare expression levels of core circadian components in fly heads; an average of six timepoints±s.e. in LD conditions (ZT 2, 6, 10, 14, 18, 22) were analysed. ( b ) The levels of pre-mRNA and mRNA of core clock components were measured by real-time PCR (RT-PCR) from a mixture of six circadian time points and scaled using an equimolar mixture of the PCR products to obtain absolute measurements between the different mRNAs or pre-mRNAs in each sample (mean±s.e. ; three biological replicas). As the values in each sample (pre-mRNA and mRNA) are normalized, the pre-mRNA/mRNA ratio is relative, not absolute (see methods for details). ( c ) RT-PCR measurements of transcriptional (grey) and steady state (black) levels of Clk and tim . Transcriptional/pre mRNA transcripts were detected using primers for intronic sequences of the genes, whereas steady-state/mature mRNAs were detected using primers flanking two exons. Expression was normalized to RP49 and rpS18. Representative experiment of three repeats is shown. ( d ) RT-PCR results presenting the ratio of mRNA bound to oligo-dT beads versus unbound mRNA. Data pooled from a mixture of six time points (mean±s.e. ; three biological replicates). ( e ) A Drosophila fly wing system was developed to monitor circadian gene mRNA expression levels (normalized to RP49 at ZT5, 17). Clk and tim levels cycle with the expected phase. The measurements were performed in triplicates for each time point using the Canton-S strain. ( f ) RT-PCR mRNA half-life measurements for Clk and cry mRNAs from fly wings treated with actinomycin D in five different time points (0–4 h after actinomycin D exposure, 12 h light/12 h dark conditions,mean±s.e. ; three biological replicates). See also Supplementary Fig. 1 . Full size image To determine whether the low mRNA levels are due to low transcription and/or high post-transcriptional control, we estimated the extent of Clk post-transcriptional regulation by comparing the ratio of pre-mRNA with steady-state mRNA using quantitative scaled RT-PCR. This comparison revealed that Clk as well as vri are under very strong post-transcriptional regulation ( Fig. 1b ). This finding is in agreement with calculations made using previously published data comparing the signal obtained from nascent mRNA with steady-state mRNA [41] ( Supplementary Fig. 1c ). Additional lines of evidence also support strong Clk post-transcriptional regulation. For example, we observed no difference between the temporal profiles of mature and pre-mRNAs encoding CLK, suggesting that Clk is a very short-lived mRNA ( Fig. 1c ). A delay, such as that observed in the profiles for tim mature and pre-mRNAs ( Fig. 1c ), indicates a longer mRNA half-life. Clk mRNA binds weakly to oligo-dT beads ( Fig. 1d ), likely reflecting a short polyA-tail [43] and strongly binds to the miRNA-effector protein AGO1 demonstrating miRNA-mediated regulation of this mRNA [32] . To determine whether Clk post-transcriptional regulation is at least partially due to rapid mRNA turnover, we estimated the Clk mRNA half-life in an oscillating system. As Drosophila cells in culture do not exhibit circadian oscillations and mRNA half-lives cannot be easily measured in living flies, we first examined whether fly-wing cultures could be used for mRNA measurements and estimation of mRNA half-lives. These cultures are widely utilized to monitor circadian rhythms with luciferase reporters [17] , [44] but have never been validated for mRNA measurements. We measured the amounts of Clk and tim mRNAs at two different time points in cultured wings. As observed in fly heads and brains, Clk and tim mRNAs displayed oscillations with opposite phase (high levels in the morning and night respectively; Fig. 1e ). We then determined the half-life of Clk and cry mRNAs by treating wings with the transcriptional inhibitor actinomycin D. The Clk mRNA half-life was very short ( ∼ 0.5 h), considerably shorter than the half-life of cry mRNA (half-life ∼ 4 h, Fig. 1f ), another circadian mRNA that oscillates with a similar phase. Clk 3′ UTR sets a threshold for CLK-driven transcription To study the functional significance of the short Clk mRNA half-life, we utilized Drosophila S2 cells, which do not express endogenous Clk mRNA or protein [45] . We co-transfected these cells with two different fluorescent reporters, both under the control of the copper-inducible metallothionein (MT) promoter, harbouring either a control or a Clk 3′ UTR ( Fig. 2a ). These reporters do not respond to transcriptional feedback (by VRI) and hence only evaluate the effect of the 3′ UTR. Expression from the reporter with the Clk 3′ UTR was significantly lower than that from control reporters, demonstrating that this 3′ UTR is strongly regulated also in S2 cells ( Fig. 2b ). Importantly, the Clk 3′ UTR rendered the reporter insensitive to increasing levels of transcription at low concentrations of inducer ( Fig. 2b , inset), suggesting a suppression/threshold mechanism to prevent leaky Clk expression from stochastic transcription events. 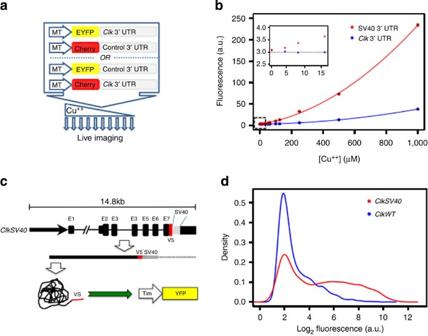Figure 2:Clk3′ UTR establishes a threshold for CLK-driven transcription (a) Schematics of the system for monitoring post-transcriptional regulation in singleDrosophilaS2 cells. (b) Mean fluorescent levels of S2 cell population expressing theClkandSV40 3′ UTRfluorescent reporters at different copper levels. The inset in the left represents a closer view of the signal at low copper concentrations (0–15 μM). Cyan fluorescent protein (CFP) expressed from a pAc-CFP plasmid was utilized as transfection control. (c) Schematics of theClkSV40andtim-YFP constructs. (d) Histogram representing the intensity of signal due to thetim-YFP reporter on transfection withClkSV40orClkWTplasmids. See alsoSupplementary Fig. 2. Red fluorescent protein (RFP) expressed from a pAc-RFP plasmid was utilized as a transfection control. Figure 2: Clk 3′ UTR establishes a threshold for CLK-driven transcription ( a ) Schematics of the system for monitoring post-transcriptional regulation in single Drosophila S2 cells. ( b ) Mean fluorescent levels of S2 cell population expressing the Clk and SV40 3′ UTR fluorescent reporters at different copper levels. The inset in the left represents a closer view of the signal at low copper concentrations (0–15 μM). Cyan fluorescent protein (CFP) expressed from a pAc-CFP plasmid was utilized as transfection control. ( c ) Schematics of the ClkSV40 and tim -YFP constructs. ( d ) Histogram representing the intensity of signal due to the tim -YFP reporter on transfection with ClkSV40 or ClkWT plasmids. See also Supplementary Fig. 2 . Red fluorescent protein (RFP) expressed from a pAc-RFP plasmid was utilized as a transfection control. Full size image To study the functional significance of the rapid Clk mRNA turnover in the context of the normal gene regulation, we generated a 14.5-kilobase (kb) Clk construct that includes all known Clk coding and regulatory sequences but also carries a SV40 3′ UTR inserted immediately downstream the open reading frame ( ClkSV40 ; Fig. 2c ). We transfected ClkSV40 or ClkWT (same transgene but carrying the wild-type Clk 3′ UTR [32] ) into Drosophila S2 cells along with a newly generated tim -YFP reporter ( tim promoter driving the expression of YFP; tim is a direct CLK-CYC target). The ClkWT construct did not detectably activate expression of the tim -YPF reporter, indicating very low CLK expression (most cells show only background fluorescence; Fig. 2d , blue line). In contrast, the presence of the ClkSV40 construct significantly increased tim -YFP levels compared with YFP levels in the presence of the ClkWT construct ( Fig. 2d ; compare mean ClkWT =15.9 with mean ClkSV40 =127). Importantly, tim -YFP reporter levels were highly variable among ClkSV40 -transfected cells, suggesting that the Clk 3′ UTR not only decreases Clk mRNA levels but makes them more uniform. Clk 3′ UTR prevents leaking CLK activity in the brain To extend these observations, we generated transgenic flies carrying the ClkSV40 transgenes. These flies express a V5 tag fused to the CLK C-terminus to allow the identification of the encoded mRNAs and proteins ( Fig. 2c ). We examined flies with the ClkWT or ClkSV40 transgene in a wild-type Clk genetic background ( ClkWT or ClkSV40 flies, respectively). Like the endogenous Clk gene, the ClkWT transgene was under tight post-transcriptional control: the mRNAs expressed from the transgene were strongly associated with AGO1 and bound poorly to oligo-dT beads ( Fig. 3a, b ). In contrast, ClkSV40 mRNAs did not associate with AGO1 and bound strongly to oligo-dT beads ( Fig. 3a, b ). This indicates that Clk post-transcriptional regulation is directed predominantly if not exclusively by the 3′ UTR. 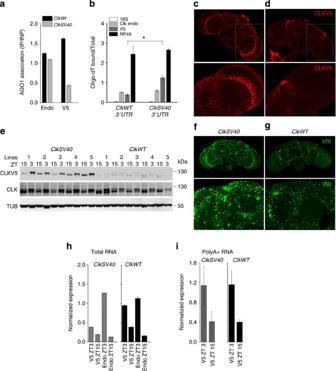Figure 3:ClkSV40flies express a stable mRNA that generates ectopic clock cells (a) AGO1 binding to endogenous genomicClkmRNA orClkV5fromClkWTorClkSV40transgenic fly heads (measured by RT-PCR, ratio of IP vs input is shown, one representative experiment out of three is presented). (b) RT-PCR results showing the ratio ofClkmRNA bound versus unbound- to oligo-dT beads inClkWTandClkSV40fly heads (*P<0.036, studentt-test; mean±s.e.n=6 for each genotype, average of five independent insertions of these transgenes were plotted). (c,d) Immunofluorescence (IF) analysis of (c)ClkSV40or (d)ClkWT Drosophilabrains using an anti-V5 antibody (lower panel represents magnification of rectangle area). (e) Expression levels of CLKV5, total CLK and tubulin proteins determined by western blot analysis of head lysates fromClkWTorClkSV40flies (five independent insertions for each transgene). The shown experiment is one out of four representative experiments. (f,g) Immunofluorescence analysis of (f)ClkSV40or (g)ClkWT Drosophilabrains using an anti-VRI antibody. (h,i)ClkV5and endogenousClkmRNAs levels fromClkSV40andClkWTfly heads determined by RT-PCR from (h) total RNA and (i) polyA+-selected RNA (for each time point, the average of five independent insertions for each transgene is plotted). See alsoSupplementary Movies 1and2. Figure 3: ClkSV40 flies express a stable mRNA that generates ectopic clock cells ( a ) AGO1 binding to endogenous genomic Clk mRNA or ClkV5 from ClkWT or ClkSV40 transgenic fly heads (measured by RT-PCR, ratio of IP vs input is shown, one representative experiment out of three is presented). ( b ) RT-PCR results showing the ratio of Clk mRNA bound versus unbound- to oligo-dT beads in ClkWT and ClkSV40 fly heads (* P <0.036, student t -test; mean±s.e. n =6 for each genotype, average of five independent insertions of these transgenes were plotted). ( c , d ) Immunofluorescence (IF) analysis of ( c ) ClkSV40 or ( d ) ClkWT Drosophila brains using an anti-V5 antibody (lower panel represents magnification of rectangle area). ( e ) Expression levels of CLKV5, total CLK and tubulin proteins determined by western blot analysis of head lysates from ClkWT or ClkSV40 flies (five independent insertions for each transgene). The shown experiment is one out of four representative experiments. ( f , g ) Immunofluorescence analysis of ( f ) ClkSV40 or ( g ) ClkWT Drosophila brains using an anti-VRI antibody. ( h , i ) ClkV5 and endogenous Clk mRNAs levels from ClkSV40 and ClkWT fly heads determined by RT-PCR from ( h ) total RNA and ( i ) polyA + -selected RNA (for each time point, the average of five independent insertions for each transgene is plotted). See also Supplementary Movies 1 and 2 . Full size image To address the ectopic and variable expression issue suggested by the S2 cells experiments, we assayed the expression of CLKV5 protein by immunohistochemistry. In ClkWT flies, expression of CLKV5 was restricted to the normal pattern (approx. 150 circadian neurons [2] ). In ClkSV40 flies, however, there was widespread expression of CLKV5 throughout the brain ( Fig. 3c, d ). Importantly, this ectopic expression was observed in five independent insertions of the ClkSV40 transgene and in none of the four ClkWT insertions that we tested ( Supplementary Fig. 2a ). Moreover, ClkSV40 fly heads contained significantly higher levels of V5-tagged CLK than ClkWT heads as determined by western blot ( Fig. 3e ). We assume that this increase is due to the presence of the ectopic circadian cells in the brain. To determine whether this ectopic expression also generated ectopic CLK-driven transcription, we analysed levels of two CLK-transcriptional targets: VRI and TIM. Immunocytochemistry using anti-VRI and anti-TIM antibodies revealed a massive increase in the number of VRI- and TIM-positive cells in ClkSV40 compared with ClkWT fly brains ( Fig. 3f,g and Supplementary Fig. 2a,b ; also see Supplementary Movies 1 and 2 for 3D visualization of VRI-positive cells in brains of ClkWT and ClkSV40 flies). To rule out the possibility that CLK ectopic expression is due to enhanced transcription mediated by the introduction of the SV40 sequence, we compared ClkV5 mRNA levels between ClkWT and ClkSV40 fly heads at two different times of the day. Surprisingly mRNA levels from the ClkSV40 transgene were even lower than those from the ClkWT transgene, demonstrating that the higher levels of CLK in ClkSV40 flies are not due to an increase in Clk transcription ( Fig. 3h , compare levels of V5-tagged Clk mRNAs). The substantial differences in the levels of CLKV5 protein ( Fig. 3e ) indicate that the Clk 3′ UTR also contributes to Clk translational regulation. This lack of a transcriptional effect was confirmed by examining the levels of V5-tagged Clk polyA + mRNAs, which were similar in flies that expressed the ClkWT and the ClkSV40 transgenes ( Fig. 3i ). ClkSV40 flies have abnormal and variable circadian behaviour To test the importance of the Clk 3′ UTR on circadian behaviour, we assessed locomotor activity rhythms in ClkWT and ClkSV40 flies. In flies with one copy of ClkWT , we observed a slightly shortened circadian period and little effect on the overall rhythm strength ( Fig. 4a and Supplementary Fig. 3a ) as previously described [28] . However, in flies with one copy of the ClkSV40 transgene, we observed a slightly more pronounced shortening of the circadian period, which was accompanied by a higher proportion of arrhythmic flies ( Fig. 4a and Supplementary Fig. 3a ). Interestingly, there was also high variability among the nine tested ClkSV40 fly insertion lines ( Fig. 4a and Supplementary Fig. 3a ). Moreover, a subpopulation of ClkSV40 rhythmic flies displayed atypical locomotor activity rhythms after a few days in constant darkness (for example, variable and in some cases split behaviour; Fig. 4b, c and Supplementary Fig. 3a ). 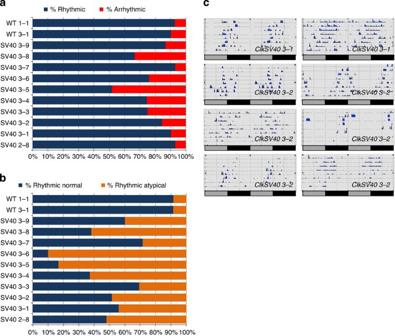Figure 4:ClkSV40flies display variable circadian behaviour (a) Bar graph summarizing the behavioural analyses ofClkWTandClkSV40flies. Each row and set of numbers (for example, 1–1) represents a strain with an independent insertion of the wild-type (ClkWT) or SV40 (ClkSV40) transgene. In all cases flies carry one extra copy of theClkgene (eitherClkWTorClkSV40) in a wild-type background. Flies were classified as rhythmic or arrhythmic in the first 5 days in constant darkness using the Behavioural toolbox44. (b) Classification of rhythmic flies as normal and atypical. The classification was done manually after 10 days in constant darkness. (c) Examples of individualClkSV40flies displaying atypical circadian behaviour. See alsoSupplementary Figs 3 and 4. Figure 4: ClkSV40 flies display variable circadian behaviour ( a ) Bar graph summarizing the behavioural analyses of ClkWT and ClkSV40 flies. Each row and set of numbers (for example, 1–1) represents a strain with an independent insertion of the wild-type ( ClkWT ) or SV40 ( ClkSV40 ) transgene. In all cases flies carry one extra copy of the Clk gene (either ClkWT or ClkSV40 ) in a wild-type background. Flies were classified as rhythmic or arrhythmic in the first 5 days in constant darkness using the Behavioural toolbox [44] . ( b ) Classification of rhythmic flies as normal and atypical. The classification was done manually after 10 days in constant darkness. ( c ) Examples of individual ClkSV40 flies displaying atypical circadian behaviour. See also Supplementary Figs 3 and 4 . Full size image The variable behaviour observed in ClkSV40 flies could be due to higher CLK levels, higher CLK-driven transcription in circadian cells or ectopic circadian gene expression. Importantly, we found no correlation between the number of ectopic VRI-expressing cells and the behavioural defects ( Supplementary Fig. 3b ). We then carefully quantified CLKV5 levels in flies carrying ClkWT and ClkSV40 transgenes using immunostaining. Surprisingly, and despite the overall difference in total protein levels and the larger number of CLKV5-positive cells ( Supplementary Fig. 4a ), there were no significant differences in the CLKV5 protein level per cell between ClkWT and ClkSV40 flies ( Supplementary Fig. 4b ). In contrast, we observed a strong effect on the levels of VRI, which was expressed in more cells and was also significantly upregulated on a per cell basis in ClkSV40 compared with ClkWT flies ( Supplementary Fig. 4c , d). VRI and CLK form a well->characterized transcriptional feedback loop: CLK is a strong transcriptional activator of vri , and VRI is the only known repressor of Clk transcription. Therefore, we surmised that the similar CLK protein levels per cell arise from very different levels of Clk transcription (high in ClkWT and low in ClkSV40 ) due to feedback transcriptional regulation by VRI. We assume that in steady state, in ClkSV40 flies CLK activity per cell is slightly higher than that in ClkWT flies, which could explain the increased levels of VRI as well as the slightly shorter period observed in these flies. A mathematical model of the CLK-VRI feedback loop It has been previously suggested that post-transcriptional control (for example, by miRNAs) could be used to diminish variability in biological systems [46] , [47] , [48] , [49] , [50] , [51] . In this context, we speculate that the high-transcriptional/high-turnover Clk profile stabilizes the circadian system by minimizing the consequences of transcriptional noise and/or by allowing rapid transcriptional feedback control. To evaluate this hypothesis, we formulated a mathematical model for uncovering factors that could modulate noise in the levels of Clk (see Supplementary Methods ). Interestingly, our model predicts that for a given target level of CLK protein, increasing the rate of Clk transcription while increasing the rate of mRNA degradation is an effective way of decreasing noise in the system ( Supplementary Fig. 5 ). As stated above, the levels of CLK per cell are similar in ClkWT and ClkSV40 flies; however, due to the strong post-transcriptional regulation provided by the Clk 3′ UTR, the same levels of protein are achieved by much lower transcriptional activity of the Clk promoter in ClkSV40 flies. In agreement with the established inverse relationship between transcriptional levels and noise [52] , [53] , [54] , [55] , our model predicted that in ClkSV40 flies CLK-driven activity would be more sensitive to transcriptional noise and hence more variable. Clk is involved in the development of the circadian neurons as well as in the control of accurate circadian transcription. Therefore, our model predicts that ClkSV40 flies might display stochastic development of the circadian neurons, which should be accompanied by random/variable circadian transcription. Decanalized development of pacemaker cells in ClkSV40 flies To test these possibilities, we first determined whether ClkSV40 flies show developmental abnormalities in the main pacemaker cells, the pdf -expressing neurons or LNvs. PDF is expressed in eight neurons in each brain lobe [18] . Most (69 out of 70) examined ClkWT brain hemispheres had eight canonical LNvs per brain lobe ( Fig. 5a ). However, flies from three independent insertions of the ClkSV40 transgene had brains with more than eight pdf ->expressing cells ( Fig. 5a–d ). Interestingly, the number of pdf -expressing cells varied between brains in these three ClkSV40 insertions. In particular, one of the lines had between eight and fourteen pdf ->expressing cells per brain hemisphere ( Fig. 5a–d ; see Supplementary Movies 3 and 4 for 3D visualization of pdf -positive cells in brains of ClkWT and ClkSV40 flies). Although these cells resemble sLNvs due to their smaller size and lower intensity ( Supplementary Fig. 6a,b ), we did not detect them in larvae brains, suggesting that they develop later than canonical sLNvs. In contrast, we found that most brains of ClkSV40 pupae had many additional pdf ->expressing cells ( Fig. 5e and Supplementary Fig. 7a,b ). Interestingly, we found that most ClkSV40 pupae brain hemispheres have larger number of pdf ->expressing cells than adults from the same strain (see Supplementary Fig. 7b ), suggesting that some of the additional pdf ->expressing cells might die or lose pdf expression later in development (or after eclosion). 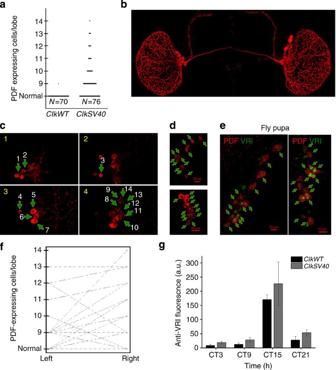Figure 5: Stochastic development of the circadian system inClkSV40flies (a) Number of PDF-positive cell bodies inClkWTandClkSV40brains. Data are from theClkSV40(2–8) andClkWT(1–1) fly strains. (b) Representative example of aClkSV40fly brain in which the position of extrapdf-expressing cells can be visualized. (c) Representative example of aClkSV40fly brain in which 14pdf->expressing cells were observed in one of the brain hemispheres.Z-stack of three images (each taken every 1 μm). Numbers in the upper left corner of each picture indicate the relative position of theZ-stack. Arrows indicate the position of thepdf->expressing cells. (d)Z-stack (maximal projection) of two brain hemispheres ofClkSV40flies immunostained for PDF showing the number ofpdf-expressing cells (13 and 12 for the top and bottom brain hemispheres respectively). Arrows indicate the position of thepdf->expressing cells. Red scale bar indicates 10 μm. (e)Z-stack (maximal projection) of two brains ofClkSV40 pupaeimmunostained for PDF (in red) and VRI (in green) showing the number ofpdf-expressing cells (14 and 15 for the left and right images respectively). Arrows indicate the position of thepdf->expressing cells. Red scale bar indicates 10 μm. (f) Comparison of left and right hemispheres inClkWTandClkSV40flies based on PDF immunofluorescent staining. (g) Brain-to-brain variation in the levels of VRI (measured by IF) protein in the sLNvs at 4 time points (day 10 in DD), inClkSV40(line 2–8, red) andClkWT(line 1–1, black) flies. See alsoSupplementary Figs 5–8Supplementary Movies 3and4. Figure 5: Stochastic development of the circadian system in ClkSV40 flies ( a ) Number of PDF-positive cell bodies in ClkWT and ClkSV40 brains. Data are from the ClkSV40 (2–8) and ClkWT (1–1) fly strains. ( b ) Representative example of a ClkSV40 fly brain in which the position of extra pdf -expressing cells can be visualized. ( c ) Representative example of a ClkSV40 fly brain in which 14 pdf ->expressing cells were observed in one of the brain hemispheres. Z -stack of three images (each taken every 1 μm). Numbers in the upper left corner of each picture indicate the relative position of the Z -stack. Arrows indicate the position of the pdf ->expressing cells. ( d ) Z -stack (maximal projection) of two brain hemispheres of ClkSV40 flies immunostained for PDF showing the number of pdf -expressing cells (13 and 12 for the top and bottom brain hemispheres respectively). Arrows indicate the position of the pdf ->expressing cells. Red scale bar indicates 10 μm. ( e ) Z -stack (maximal projection) of two brains of ClkSV40 pupae immunostained for PDF (in red) and VRI (in green) showing the number of pdf -expressing cells (14 and 15 for the left and right images respectively). Arrows indicate the position of the pdf ->expressing cells. Red scale bar indicates 10 μm. ( f ) Comparison of left and right hemispheres in ClkWT and ClkSV40 flies based on PDF immunofluorescent staining. ( g ) Brain-to-brain variation in the levels of VRI (measured by IF) protein in the sLNvs at 4 time points (day 10 in DD), in ClkSV40 (line 2–8, red) and ClkWT (line 1–1, black) flies. See also Supplementary Figs 5–8 Supplementary Movies 3 and 4 . Full size image Interestingly, we observed that the two lobes of individual flies carrying ClkSV40 transgenes flies did not necessarily have the same number of pdf ->expressing neurons, demonstrating that the number of these neurons is variable in the absence of Clk post-transcriptional regulation ( Fig. 5b,f ). We observed the same phenomenon in pupae of ClkSV40 flies ( Supplementary Fig. 7c ) demonstrating that this asymmetry is established during development. To determine whether Clk 3′ UTR also diminishes variability in daily CLK-driven transcription within adult flies, we determined VRI levels throughout the day in flies carrying ClkWT or ClkSV40 transgenes. We focused on one ClkWT (1-1) and one ClkSV40 (2–8) insertions of the transgenes. To minimize the effects of an endogenous WT Clk gene, we performed the experiment in the background of the Clk hypomorphic mutant Clk AR (ref. 29 ). In these transgenic lines, the ClkWT transgene rescued the arrhytmicity of the Clk AR mutation much more effectively (>75%) than the ClkSV40 transgene (<40%). Therefore, we stained ClkWT ; Clk AR and ClkSV40 ; CLK AR flies for VRI and PDF at four different circadian time points after 8 days in constant darkness (DD8). We focused on the sLNvs, which display strong protein oscillations in constant darkness [37] . Whereas ClkWT ; Clk AR flies displayed robust VRI protein oscillations and little brain-to-brain variability, ClkSV40 ; Clk AR flies expressed higher and more variable VRI levels with a significant number of flies showing inappropriate VRI staining at the early circadian time points (CT3 and CT7; Fig. 5g and Supplementary Fig. 8 ). A role of bantam in the development of circadian neurons We recently showed that the miRNA bantam regulates the Clk 3′ UTR, at least in Drosophila S2 cells [32] . Hence, we decided to define whether this regulation is key to the deterministic development and maintenance of the circadian neuronal network. For doing so, we examined by immunocytochemistry the number and intensity of circadian neurons (VRI- and PDF-positive cells) in flies carrying a Clk transgene with deletion of the putative bantam binding sites ( ClkΔban [32] ). Indeed, and similarly to ClkSV40 flies, ClkΔban displayed ectopic expression of VRI across the fly brain ( Fig. 6a ). In addition, ClkΔban showed variable and increased number of pdf ->expressing cells ( Fig. 6b,c ). Importantly, and as in ClkSV40 flies, we did not observe a correlation between the numbers of pdf ->expressing cells in each hemisphere of individual fly brains ( Fig. 6d ). These results demonstrate the importance of the bantam binding sites in the Clk 3′ UTR for normal development of the pdf ->expressing cells. Interestingly, we found that some of these brains also have heterogeneous VRI expression in the PDF-positive cells. For example, we found brains in which VRI expression differs or is even absent in some of the PDF-positive cells (that is, see Fig. 6b ). We observed a similar phenomenon in ClkSV40 pupae (see Fig. 5e and Supplementary Fig. 6a ). This strongly suggests that CLK activity is variable across circadian neurons within the same brain. 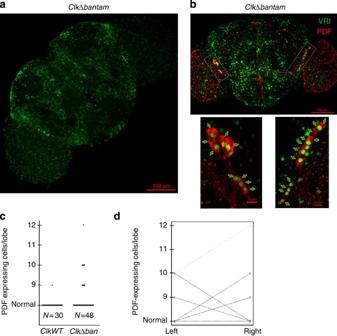Figure 6: Deletion of thebantambinding sites on theClk3′ UTR leads to stochastic development of thepdf->expressing cells (a) Immunofluorescence (IF) analysis of a representativeClkΔban(3–7)Drosophilabrain using an anti-VRI antibody. Flies were collected and dissected at ZT15. (b) Representative example of aClkΔbanfly brain in which 21 LNvs cells were observed, 9 in one hemisphere and 12 in the other (top panel). Lower panel represents magnification of rectangle area. Of the 12 PDF-positive cell bodies in the right hemisphere: 9 cells are VRI positive, one cell display low intensity of VRI immunostaining and 2 cells are VRI negative. In the left hemisphere of the brain, 9 PDF-positive cells are observed: 8 cells are VRI positive and one cell displays low intensity of VRI immunostaining. Flies were collected and dissected at ZT15. Arrows indicate the position of each PDF-positive cell. (c) Number of PDF-positive cell bodies inClkWTandClkΔbanbrains. Data are taken from theClkΔban(3–7) andClkWT(1–1) fly strains. (d) Comparison of left and right hemispheres inClkWTandClkΔbanflies. Figure 6: Deletion of the bantam binding sites on the Clk 3′ UTR leads to stochastic development of the pdf ->expressing cells ( a ) Immunofluorescence (IF) analysis of a representative ClkΔban (3–7) Drosophila brain using an anti-VRI antibody. Flies were collected and dissected at ZT15. ( b ) Representative example of a ClkΔban fly brain in which 21 LNvs cells were observed, 9 in one hemisphere and 12 in the other (top panel). Lower panel represents magnification of rectangle area. Of the 12 PDF-positive cell bodies in the right hemisphere: 9 cells are VRI positive, one cell display low intensity of VRI immunostaining and 2 cells are VRI negative. In the left hemisphere of the brain, 9 PDF-positive cells are observed: 8 cells are VRI positive and one cell displays low intensity of VRI immunostaining. Flies were collected and dissected at ZT15. Arrows indicate the position of each PDF-positive cell. ( c ) Number of PDF-positive cell bodies in ClkWT and ClkΔban brains. Data are taken from the ClkΔban (3–7) and ClkWT (1–1) fly strains. ( d ) Comparison of left and right hemispheres in ClkWT and ClkΔban flies. Full size image Here we found that the circadian master regulator Clk is under very strong post-transcriptional control. One consequence of this tight control is the creation of a threshold-like regulation that inhibits ectopic expression of Clk and CLK-transcriptional targets. Indeed, flies devoided of this regulation have more circadian cells in the brain and aberrant and variable circadian rhythms. Interestingly, in these flies, the levels of CLK on a per cell basis are not altered compared with flies with wild-type CLK, suggesting that the main role of Clk post-transcriptional regulation is to limit the variability of CLK activity rather than CLK protein levels. Moreover, we observed an increase in the number of pdf ->expressing cells in ClkSV40 flies and pupae. To understand these results, we formulated a mathematical model of the circadian CLK-VRI feedback loop. Our model predicts that Clk post-transcriptional control diminishes the noise in this transcriptional feedback loop. Indeed, we found that in ClkSV40 flies there were not only more pdf ->expressing cells, but also that their numbers were variable among individuals or between the two lobes of the same brain, demonstrating that in the absence of Clk post-transcriptional control LNvs development and maintenance is stochastic. Last, flies carrying Clk transgenes with mutation in the putative binding sites for the miRNA bantam also displayed stochastic number of pdf ->expressing cells between and within individuals, suggesting that the phenotypes observed in ClkSV40 flies are mediated through this miRNA. Clk is strongly regulated at the post-transcriptional level. Indicative of regulation by miRNAs, Clk mRNA is strongly bound to AGO1 and does not bind efficiently to oligo-dT beads. In addition, we observed significant differences between the CLK protein and Clk mRNA ratios in ClkWT and ClkSV40 flies (compare Fig. 3h to Fig. 3e ), which suggests that an important part of this regulation is at the translational level. Interestingly, mRNA turnover accounts at least partially for the post-translational control, as Clk mRNA is short lived when compared with other circadian mRNAs like cry ( Fig. 1f ). Therefore, Clk post-transcriptional regulation appears to be complex and redundant. Our results suggest that the Clk 3′ UTR is responsible for the decrease in CLK levels in most (if not all) cell types, likely by miRNAs. Bantam seems to have a predominant role but it might not be unique. The presence of this type of regulation is not surprising given the large amount of reports demonstrating the importance of RNA metabolism for circadian timekeeping [28] , [41] , [56] , [57] , [58] , [59] , [60] . The general assumption in the field is that Clk transcriptional oscillations are not essential for behavioural rhythms. This is based on the fact that the circadian behaviour of clk AR mutants can be rescued using the cry-GAL4 driver and a UAS- Clk transgene [29] and that there are negligible effects on expression of CLK under the per or tim promoters (ARK flies [21] ). However, the same UAS- Clk transgene expressed under control of other gal4 drivers like tim-gal4 leads to developmental lethality [29] and the behavioural deficits of Clk AR mutants are not rescued by Clk ARK transgenes (our own unpublished observation). Moreover, addition of extra Clk gene copies leads to a copy-number-dependent shortening of the period [28] , demonstrating that CLK levels cannot be regulated solely at the post-translational level. Interestingly, the ARK transgenes carry a per 3′ UTR, which is strongly regulated post-transcriptionally (our unpublished data). This could explain why flies carrying this transgene are rhythmic in a wild-type background. Our S2 cells and fly brains experiments demonstrate a key role of Clk 3′ UTR in avoiding ectopic CLK-driven transcriptional activity. Moreover, these results suggest that the Clk 3′ UTR is necessary for establishment of a threshold for meaningful Clk mRNA expression. This type of threshold might be important not only in circadian cell determination but also to prevent stochastic or random pulses of CLK-driven activity that could alter or shift the circadian clock. miRNA-mediated thresholding of master developmental regulators has been previously demonstrated for the miR-9a/ senseless [61] and for the miR-263a/ hid pairs [62] . We believe that our failure to detect signal from the Clk 3′ UTR reporters is not related to a sensitivity issue. This is based on our observation of the abnormally high number of circadian cells in the brains of ClkSV40 flies, which demonstrates that the threshold has a biological meaning. Our work demonstrates a central role for Clk in the development of the pdf ->expressing LNvs cells, as three of the fly lines with ClkSV40 insertions as well as ClkΔban flies display larger number of LNvs than observed in wild-type brains. Although this work constitutes the first report of flies with more than 16 LNvs per brain, a previous report suggests that Clk affects the development of these cells: Clk and cyc mutants have reduced numbers of LNvs, and Clk can activate (albeit weakly) a pdf-luciferase reporter [31] . From our results it is not clear whether these cells are part of the neuronal circadian network or whether their development and maintenance is independent. Indeed, the transgenic line with the largest number of extra LNvs ( SV40 2–8) was fairly rhythmic at the behavioural level, suggesting that these extra cells do not markedly influence the timekeeping process, at least early in constant darkness. The abnormal behaviour cannot be explained neither by the presence of additional VRI-expressing cells, as we see no correlation between the number of them and any of the behavioural anomalies ( Supplementary Fig. 3b ). We favour the possibility that the behavioural defects are due to stochastic changes in CLK-driven transcription. Stochastic variation in CLK-driven transcription could also explain the brain-to-brain variation in VRI levels in ClkSV40 flies and the observed variations in VRI levels between pdf ->expressing cells within the same brain in the ClkSV40 pupae and ClkΔban fly brains (that is, see Figs 5e and 6b bottom, respectively). Moreover, we observed that ClkSV40 pupae have generally larger numbers of extra LNvs, suggesting that many of these cells might lose pdf expression during adulthood (as we did not observed high levels of lethality in ClkSV40 flies). We believe that in the future and given the advances in CRISPR technology, it would be interesting to repeat some of the experiments in flies in which the deletion the 3′-UTR is in the endogenous Clk locus. Our results suggest that the main role of Clk post-transcriptional control is to limit the variability in CLK activity rather than to control the total levels of CLK. This is based on the fact that the levels of CLK per cell were not altered in ClkSV40 flies despite the large increase in the total number of CLK-positive cells. We argue that the normal CLK levels in individual cells are due to an increase in VRI levels that reduce Clk transcription and hence total CLK levels (see model in Fig. 7 ). Indeed, heads of ClkSV40 flies have lower levels of ClkV5 mRNA than do ClkWT flies ( Fig. 3h ) despite much higher protein levels ( Fig. 3e ). Therefore, our data suggest that the main difference between ClkWT and ClkSV40 flies is that the latter produce CLK by a low transcription/low degradation rather than the high transcription/high degradation profile observed in wild-type flies ( Fig. 7 ). We speculate that the increase in VRI levels keeps the overall levels of CLK per cell constant. In contrast, the low transcription/low turnover Clk mRNA profiles observed in ClkSV40 flies lead to more random, less fixed levels of Clk mRNA and protein ( Fig. 7 ). We can then imagine a model in which under wild-type conditions (either no Clk transgene or one copy of the ClkWT transgene) stochastic pulses of Clk transcription in non-circadian neurons are filtered by the transcriptional threshold and do not lead to the development of circadian cells ( Fig. 7 ). This is essential during development as well as in adult animals, as ectopic clocks in the fly brain are dependent on continuous expression of Clk [63] . In theory, Clk post-transcriptional control could help stabilize CLK-driven transcription in the circadian cells both by thresholding and by diminishing cell-to-cell variability in CLK-driven oscillations ( Fig. 7 ). 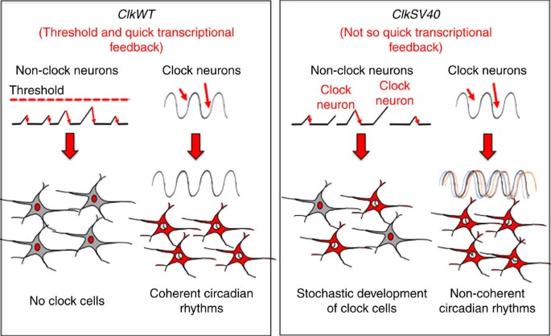Figure 7: Role ofClkpost-transcriptional regulation in clock and non-clock neurons Small red arrows represent random or environmentally driven fluctuations inClkgene expression. Figure 7: Role of Clk post-transcriptional regulation in clock and non-clock neurons Small red arrows represent random or environmentally driven fluctuations in Clk gene expression. Full size image In sum, here we found that post-transcriptional control of a master transcriptional regulator provides an efficient mechanism that assures canalized development and that stabilizes a transcriptional network during development and in adult animals. The role of post-transcriptional control in stabilizing the activities and levels of key activators of systems based on feedback loops has been previously proposed [46] , [47] , [51] , but to the best of our knowledge, our work constitutes the first theoretical and experimental example of this control principle. Fly strains The CantonS (CS) strain used as wild type is CSIso3H (Bloomington Stock Centre, Indiana). Clk AR mutants were described [29] . ClkSV40 flies were constructed by injecting ClkSV40 transgene into yw embryos (service provided by Best Gene). ClkΔban flies were described [32] . Analysis of gene expression by real-time PCR Total RNA was prepared from adult fly heads using TRI Reagent (SIGMA) according to the manufacturer’s protocol. RNA was DNase treated (DNaseI, NEB), and cDNA derived from this RNA (using iScript, Bio-Rad) was utilized as a template for quantitative real-time PCR performed with the C1000 Thermal Cycler Bio-Rad. The utilized primers are summarized in Supplementary Methods . mRNA values from heads were normalized to levels of mRNAs encoding ribosomal proteins RP49 and rpS18. Assessment of post-transcriptional regulation We utilized a mixture of RNA extracted at six different time points from fly heads. The three biological replicas were generated by three independent RNA extractions from each of the six time points. After extraction, the RNA was DNase treated, ethanol precipitated and retrotranscribed using iScript (Bio-Rad) with random primers. We performed real-time PCR using the diluted cDNA template and an equimolar mixture of the DNA products. This DNA mixture was utilized in experiments to determine the absolute levels of the pre-mRNA and mature mRNA. We generated this mixture by pooling equimolar concentrations of the purified PCR products. We designed two sets of primers for each gene, one intronic and one exonic. For intronic PCRs, real-time PCR was performed using the cDNA as a template, and amounts were plotted on a standard curve constructed using different concentrations of the genomic DNA as templates to normalize the different efficiencies of the primers. For each gene a pre-mRNA/mRNA ratio was calculated. The primer sequences are detailed in Supplementary Information . Three independent biological replicates were performed. Isolation of different fractions of RNAs Oligo-dT-bound fractions were isolated from total RNA using Invitrogen (dT) 25 Dynabeads following the manufacturer’s protocol. The RNA not bound was precipitated with ethanol and dissolved in RNase-free water. For quantification, the unbound fraction was normalized to histone H1 and the bound fraction to RP49. Data were obtained from a pooled mixture of six time points, and three biological replicates were performed. RNA measurements from cultured fly wings Thirty adult male Canton-S fly wings were dissected and cultured as described [64] under 12 h light/12 h dark (LD) conditions for 3 days. In mRNA half-life measurements actinomycin D was added in ZT3 (10 μg ml −1 ), wings were transferred into TRI Reagent (SIGMA) at relevant time points and mRNA was extracted. For each time point, the experiments were performed in triplicates. Plasmids To generate the tim -YFP reporter, we amplified by PCR the YFP coding sequence and the tim promoter region (760 bp from the timwt760-luciferase construct [65] ). The fragments were ligated sequentially into pBluescript. pAc-Cherry and pAc-CFP were constructed by amplifying the Cherry or CFP coding sequences by PCR and ligating these products into pAcB V5/His6 (Invitrogen). The ClkSV40 plasmid was generated through steps similar to those used to construct the ClkWT (described in [28] ) with the following modification: a fragment containing the SV40 3′ UTR sequence was amplified by PCR from pAc V5/His6 (Invitrogen) and cloned by overlap PCR, exactly downstream the stop codon, into a plasmid containing a Sph-NotI fragment derived from a plasmid containing the last portion of the Clk transgene (from position 7741779 to 7736982, pdClk 4). The Sph-NotI fragment containing the SV40 3′ UTR was re-cloned into the pdClk 4, which was then used to generate the whole ClkV5 transgene as described previously [28] . The resulting plasmid was fully sequenced. S2 cells maintenance and transfection S2 cells were maintained in 10% fetal bovine serum (Invitrogen) insect tissue culture medium (HyClone). Cells were seeded in a six-well plate. Transfection was performed using 6 μl of MIRUS transfection reagent TransIT 2,020 and 2 μg of total DNA as per the manufacturer’s instruction. For the 3′ reporter experiments, 250 ng each of pMT-Cherry and pMT-YFP reporters (one carrying the SV40 3′ UTR and one carrying the Clk 3’ UTR) were co-transfected into Drosophila S2 cells along a pAc-CFP transcriptional control. To avoid bias due to the different fluorophores, we performed the analysis comparing the levels of the same fluorescent protein under the different 3′ UTRs ( SV40 versus Clk 3′ UTR). Shown are data obtained with the Cherry reporter, but we obtained similar results when YFP reporters were compared. For the experiments to follow CLK-driven activity, we utilized 150 ng of pAcCherry, 150 ng of the tim -YFP reporter and 500 ng of the ClkWT or ClkSV40 plasmids. pBS-KS (Stratagene) was used to bring the total amount of DNA to 2 μg. High-throughput reporter expression analysis in S2 cells One day after transfection, cells were transferred to optic-suitable 96-well plates and visualized over 24 h using Scan^R high-throughput fluorescent microscope (Olympus). The intensity from the transfection control reporter (CFP for 3′ UTR and Cherry for the CLK-activity experiments), cell size and roundness were evaluated. Cherry or YFP levels were assessed only for cell populations that met intensity and cell morphology criteria. AGO-1 immunoprecipitation AGO-1 immunoprecipitations were performed as previously described [32] . The transcripts were quantified by RT-PCR using primers that exclusively identify the endogenous (endo) or the V5-tagged Clk mRNA (V5). Data are shown as ratio of immunoprecipitate to input. Immunofluorescence Male flies were entrained for at least 3 days in LD and then transferred to DD for the indicated time. Third stage larvae and last stage pupae were collected after 3 days entrainment in LD. Whole flies/larvae/pupae were collected into fixative solution, PBS 4% paraformaldehyde 0.1% Triton X-100, and incubated for 30 min at 4 °C followed by 2 h rotation at room temperature. After fixation, flies/larvae/pupae were transferred to PBS, and the brains were dissected. The brains were washed three times (PBS 0.1% Triton X-100) and transferred to blocking solution (PBS, 0.1% Triton X-100, 2% horse serum). After three washes, primary antibody solution was added and samples were incubated at 4 °C overnight. The primary antibody solution contained PBS, 0.1% Triton X-100, 2% horse serum, and 1:3,000 guinea pig anti-VRI (gift from Paul Hardin), 1:1,000 mouse anti-PDF (gift from the Justin Blau lab), 1:1,000 mouse anti-V5 (Sigma), 1:1,000 rat anti-TIM (a gift from Michael Rosbash) or 1:1,000 guinea pig anti-CLK (a gift from Paul Hardin). Brains were washed three times and then exposed to secondary antibody solution: PBS, 0.1% Triton X-100, 2% horse serum and 1:500 Alexa Fluor 488 goat anti-guinea pig (Invitrogen), 1:500 Dylight 550 donkey anti-mouse (Abcam) or 1:500 Alexa Fluor donkey anti-rat (Jackson) for 1 h in room temperature. Brains were washed three times and mounted in VECTASHIELD mounting medium (VECTOR) on microscope slides. Images were captured using a Nikon A1R confocal microscope and analysed with NIS-Elements (Nikon). Quantification of brain cell expression of V5 or VRI proteins was performed as follows: stained brains were placed between spacers to avoid pressure on the tissue. Confocal images were taken every 3 μm (on the Z axis) over the entire brain depth. Western blotting Fly heads (20 heads per sample) were collected on dry ice. Heads were homogenized in RIPA lysis buffer (50 mM Tris-HCl at pH 7.4, 150 mM NaCl, 1 mM EDTA, 1% NP-40, 0.5% sodium deoxycholate, 0.1% sodium dodecyl sulfate, and 1 mM DTT, supplemented by protease inhibitor cocktail and phosphatase inhibitors) using a motorized pestle. Head lysates were then centrifuged at top speed for 10 min. The supernatant was boiled with protein sample buffer (Bio-Rad). Samples were resolved on Criterion XT Bis-Tris gels (Bio-Rad). Antibodies used for western blotting were those described above and anti-tubulin (DM1A, SIGMA).The complete blots of Fig. 3e are provided as Supplementary Fig. 9 . Locomotor activity Male flies were monitored using trikinetics Drosophila activity monitors. Analyses were performed with a signal processing toolbox [44] . Flies were considered rhythmic if the rhythm index was >0.15 for the first 5 days in DD. Rhythmic flies after the 5-day period were followed for 5 more days and, if alive after this period, were classified as normal or atypical rhythmic by visual inspection after examination of the behavioural pattern and the MESA analysis. How to cite this article: Lerner, I. et al . Clk post-transcriptional control denoises circadian transcription both temporally and spatially. Nat. Commun . 6:7056 doi: 10.1038/ncomms8056 (2015).